Evidence for an electrostatic mechanism of force generation by the bacteriophage T4 DNA packaging motor How viral packaging motors generate enormous forces to translocate DNA into viral capsids remains unknown. Recent structural studies of the bacteriophage T4 packaging motor have led to a proposed mechanism wherein the gp17 motor protein translocates DNA by transitioning between extended and compact states, orchestrated by electrostatic interactions between complimentarily charged residues across the interface between the N- and C-terminal subdomains. Here we show that site-directed alterations in these residues cause force dependent impairments of motor function including lower translocation velocity, lower stall force and higher frequency of pauses and slips. We further show that the measured impairments correlate with computed changes in free-energy differences between the two states. These findings support the proposed structural mechanism and further suggest an energy landscape model of motor activity that couples the free-energy profile of motor conformational states with that of the ATP hydrolysis cycle. Many double-stranded DNA viruses utilize a powerful molecular motor during assembly to translocate DNA into a preformed capsid shell [1] , [2] , [3] , [4] , [5] , [6] . The motor must do significant mechanical work against forces arising from DNA-bending rigidity, electrostatic self-repulsion and entropy loss, which oppose DNA confinement [7] , [8] , [9] , [10] , [11] , [12] . Measurements of DNA packaging with optical tweezers in bacteriophages φ 29, λ and T4 show that all three motors can generate forces >50 pN, which is >20 × higher than forces generated by skeletal muscle myosin motors [1] , [13] , [14] . The motors differ in DNA translocation rates, which range from up to ~200 bp s −1 for φ 29 to up to ~2,000 bp s −1 for the T4 motor [13] , [14] , [15] . A number of studies have begun to examine the microscopic details of the motor mechanism. Measurements of single-DNA packaging dynamics of φ 29 via optical tweezers have enumerated the mechanical and chemical kinetic transitions and rate constants, step size and coordination of motor subunits [1] , [16] , [17] , [18] . Bioinformatics analyses and mutagenesis studies altering the λ and T4 motor proteins indicate the presence of several functional motifs that are homologous with the ASCE (additional strand, conserved E) superfamily of ATPases, including the DNA and RNA-translocating helicases and chromosome segregating transporters [19] , [20] , [21] . Single-molecule packaging measurements with phage λ showed that mutations in the Walker A, C-motif, Q-motif and other structurally conserved regions of the large terminase subunit cause phenotypic impairments in motor function, including reduced translocation velocity, increased pausing and slipping, and steepening of the force–velocity relationship [22] , [23] . The structure–function relationships for these motors have remained unclear due to lack of high-resolution structures, unlike the situation for other biomotors such as helicases and F1-ATPase where sophisticated structural models have been proposed [24] , [25] , [26] . The recent determination of a high-resolution X-ray structure of the T4 large terminase subunit (gp17), along with cryo-electron microscopy (EM) reconstruction of the entire prohead–motor complex, has made this system attractive for probing detailed structure–function relationships of viral DNA packaging [27] . The cryo-EM data indicates that the motor consists of a pentameric ring of gp17 subunits attached to a dodecameric ring of gp20 proteins, together forming the portal entry channel ( Fig. 1a ). gp17 was found to have globular N- and C-terminal subdomains connected by a flexible linker region. While there has been some debate regarding which subdomain binds to the portal based on studies of several different phages using multiple different techniques [28] , [29] , [30] , fitting of the gp17 crystal structure into the cryo-EM density of the prohead-motor complex suggests that it is the N-terminal subdomain [27] . Comparisons also revealed two distinct conformations: a ‘compact’ state seen in the X-ray structure of the gp17 monomer in which the N- and C-terminal domains are in close contact, and an ‘extended’ state, seen in the cryo-EM structure of packaging complexes in which the N- and C-terminal domains are separated by ~7 Å (previously referred to as ‘tensed’ and ‘relaxed’ states, respectively) [27] . 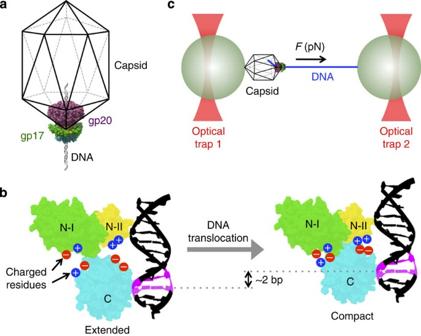Figure 1: Schematic overview of the T4 packaging motor structure and the single-molecule measurement technique. (a) The T4 packaging motor consists of concentric rings of gp17 (motor) and gp20 (portal) proteins at the special fivefold vertex of the viral capsid. (b) Structural data indicate that gp17 can adopt extended (left) and compact states (right). The X-ray structure shows a large interface between the N-terminal (composed of two sub-regions, N-I and N-II) and C-terminal globular subdomains containing pairs of apparently aligned complimentarily charged residues. The electrostatic force model27proposes that attractive interactions between these residues generates the force during a conformational change from the extended to the compact state that translocates the DNA into the capsid in steps of ~2 bp. (c) Dual optical tweezers are used to measure the packaging of single DNA molecules into single capsid–motor complexes under applied load forces. Figure 1: Schematic overview of the T4 packaging motor structure and the single-molecule measurement technique. ( a ) The T4 packaging motor consists of concentric rings of gp17 (motor) and gp20 (portal) proteins at the special fivefold vertex of the viral capsid. ( b ) Structural data indicate that gp17 can adopt extended (left) and compact states (right). The X-ray structure shows a large interface between the N-terminal (composed of two sub-regions, N-I and N-II) and C-terminal globular subdomains containing pairs of apparently aligned complimentarily charged residues. The electrostatic force model [27] proposes that attractive interactions between these residues generates the force during a conformational change from the extended to the compact state that translocates the DNA into the capsid in steps of ~2 bp. ( c ) Dual optical tweezers are used to measure the packaging of single DNA molecules into single capsid–motor complexes under applied load forces. Full size image Based on the two different conformations of gp17 seen in the structural data, Sun et al. [27] proposed a model for motor operation in which the DNA is translocated in ~7 Å ( ≅ 2 bp) increments by the transition of gp17 from the extended-to-compact state ( Fig. 1b ). Inspection of the interface between the domains revealed five aligned pairs of complimentarily charged residues, which led to the proposal that this transition is driven by electrostatic interactions between these charged residues across the interface that generate force to translocate the DNA into the prohead. ATP hydrolysis was proposed to regulate DNA interaction and provide energy to return gp17 to the extended state after each 2-bp DNA translocation step. We refer to this model as the ‘electrostatic force model’. Another model for T4 packaging in which the portal grips the DNA and gp17 exerts force that compresses the DNA until the portal releases it has been proposed [31] . Although many aspects of these models are not mutually exclusive, and several different packaging models describing other systems, including one based on the crystal structure of phage Sf6 large terminase gp2, have been proposed [3] , [4] , [32] , [33] , [34] , [35] , [36] , the model proposed by Sun et al. [27] is the only one to propose a detailed mechanism implicating specific residues as critical for force generation based on the atomic structure of the motor protein. Here, we examine the force-generating mechanism of the T4 motor by measurements of single DNA molecule packaging dynamics with increasing applied forces ( Fig. 1c ) and characterize the effects of mutations that alter charged residues at the interface between the N- and C-terminal subdomains identified in the crystal structure. We also carried out molecular dynamics (MD) simulations to predict free-energy difference between the extended and compact states of gp17 and effect of the residue changes. We find that computed changes in free-energy correlate strongly with measured impairments of motor function, consistent with the electrostatic force model. Our findings suggest a simple mechanochemical energy landscape picture of gp17 motor dynamics that can explain the experimental observations and simulations. Site-directed mutagenesis To investigate whether the pairs of apparently aligned, complimentarily charged residues within the domain interface observed in the gp17 crystal structure are critical to motor function, we used site-directed mutagenesis to alter these residues. 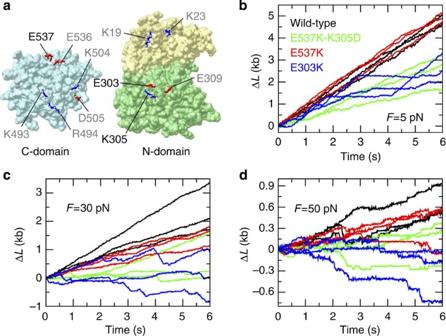Figure 2: Locations of altered charged residues and measurements of DNA packaging dynamics. (a) Open book representation of the N- and C-terminal domain interface of gp17 (PDB ID code 3CPE) displaying the charged residues studied in this work. Changes in the residues labelled in grey resulted in zero bulk packaging while those labelled in black resulted in some packaging, leading to their further study through measurements with optical tweezers. Red indicates acidic interface residues, while blue indicates basic interface residues. (b–d) Representative measurements of single DNA molecule packaging dynamics (length packaged versus time) with (b) 5 pN applied load, (c) 30 pN and (d) 50 pN. The colours indicate WT (black), E537K (red), E537K-K305D (green) and E303K (blue) gp17 motors. Figure 2a shows the locations of the mutated residues in the motor (see Supplementary Fig. 1 for additional views). We substituted these amino acids with ones with reversed charges (that is, we changed ‘+’ to ‘−’ or ‘−’ to ‘+’) to weaken the putative attractive electrostatic interactions between the N- and C-terminal subdomains proposed to generate force. In particular, six mutants with single-residue changes (K23E, E303K, K305D, E309K, K504E and E537K) and three with double-residue changes (E303K-K504E, E537K-K305D and E537K-K504E) were studied. Of these, six exhibited little or no packaging activity, as measured in bulk packaging reactions by DNase protection assays ( Supplementary Fig. 2 ). While these findings suggest that these residues play an important role in packaging it is important to note that packaging activity as assessed by only these bulk assays can exhibit impairment for multiple reasons, including failure of motor proteins to fold and assemble into active multimeric complexes, or initiate interactions with DNA. Three of the mutants (E303K, E537K and E537K-K305D) exhibited sufficient activity to permit detailed measurements of packaging dynamics using the single-molecule optical tweezers assay. Figure 2: Locations of altered charged residues and measurements of DNA packaging dynamics. ( a ) Open book representation of the N- and C-terminal domain interface of gp17 (PDB ID code 3CPE) displaying the charged residues studied in this work. Changes in the residues labelled in grey resulted in zero bulk packaging while those labelled in black resulted in some packaging, leading to their further study through measurements with optical tweezers. Red indicates acidic interface residues, while blue indicates basic interface residues. ( b – d ) Representative measurements of single DNA molecule packaging dynamics (length packaged versus time) with ( b ) 5 pN applied load, ( c ) 30 pN and ( d ) 50 pN. The colours indicate WT (black), E537K (red), E537K-K305D (green) and E303K (blue) gp17 motors. Full size image Measurements of DNA-packaging dynamics at low force We first carried out single-molecule packaging measurements using the low force-clamp technique described previously [14] . Briefly, T4 prohead–motor complexes were assembled using purified recombinant gp17, attached to microspheres via antibodies, injected into a fluid chamber containing ATP and trapped in one optical trap. DNA molecules were biotinylated at one end and attached to streptavidin-coated microspheres and trapped in a second optical trap. Packaging was initiated by bringing the two microspheres into proximity such that the motor binds to and begins reeling in the DNA, thus exerting a force that pulls the two microspheres together ( Fig. 1c ). DNA translocation was tracked using a feedback control system that held the applied load force at a constant value of 5 pN, which is low compared with the maximum force generated by the WT motor (>60 pN). Measurements were made with the three mutants and with wild-type (WT) gp17 for comparison ( Fig. 2b ). We found that E537K mutants packaged at nearly the same rate (~600 bp s −1 ) on average as WT, while E303K and E537K-K305D mutants showed a modest reduction to ~400 bp s −1 . The reductions were partly due to an increase in pausing and slipping and partly due to inherently reduced motor velocity (as shown below). These results clearly show that some of the charged residues at the interface play an important role in the DNA translocating function of the T4 motor. However, given that one mutant (E537K) exhibited no measurable change, the other two mutants exhibited only modest changes, and unexpectedly, the double mutant (E537K-K305D) did not show greater impairment, support for the electrostatic force model from these measurements alone could be considered ambiguous. High force measurements We next investigated the motor response under increasing applied loads, where the impact of changes in residues putatively involved in force generation would be expected to be greater. In our previous studies of the WT motor, high force measurements were made by holding the trap positions fixed and allowing the tension in the DNA to build up due to the shortening of the DNA tether accompanying packaging [14] . This approach is undesirable for characterizing mutants because they package DNA at slower rates, which would cause a slower build-up of force. This would lead to a bias in the comparison of the WT and different mutants, as different complexes would experience different force-loading histories. In addition, prolonged force build-up frequently leads to rapid detachment of the tethered complexes before the target force is reached, due to the DNA slipping out of the prohead or dissociation of the prohead from the antibody-coated microsphere [14] , [37] . Therefore, in the present work we implemented a new protocol in which we first packaged ~5 kb of DNA at low force (5 pN) to confirm activity, and then quickly ramped the force to a higher value and clamped it via feedback control to measure the response of the motor. Thus, all complexes, WT and mutants, were subject to the same force-loading history. Using this new protocol, force-clamp measurements were recorded at 5, 15, 30, 40, 50 and 60 pN loads. Examples of individual packaging traces are shown in Fig. 2c,d , highlighting the highly variable and stochastic nature of packaging by the gp17 motor. We also note the presence of pauses in translocation (flat regions) and slippage (negative slope) interspersed with DNA packaging episodes (positive slope). The overall trend is that velocity decreases with increasing applied load, which implies that the rate-limiting step in the mechanochemical cycle involves DNA translocation and, hence, mechanical work done by the motor against the load slows down the overall motor velocity [38] . Mutations further slow packaging and the time spent pausing and slipping also increases with increasing load and mutations. A perhaps unexpected minor feature in the data is the occurrence of a similar average packaging rate at 30 pN and 15 pN and slightly higher % time packaging at 30 pN than at 15 pN. The cause of this behaviour is not clear, but it may be related with the observation that the motors sustain the 15 pN load for much longer time (115 s, on average) than the 30 pN load (32 s, on average). We analysed ensembles of packaging trajectories to determine several averaged metrics of motor function ( Fig. 3 ). Specifically, we calculated the ‘packaging rate’, defined as the net length of DNA packaged per unit time; the ‘motor velocity’, defined as the rate of DNA translocation during episodes of packaging (that is, not including pauses and slips); and the ‘percent time spent packaging’, defined as the percentage of time packaging occurs (versus pausing or slipping). All three metrics show that the residue changes cause more severe impairment at high load than at low load. For example, the average packaging rate for mutant E303K, which was ~400 bp s −1 at 5 pN, drops below zero at forces ≥15 pN. E303K exhibits episodes of packaging, but slips so frequently that there is no net packaging. The average packaging rates for E303K and E537K-K305D, which were nearly the same at 5 pN, also exhibited a clear difference at forces ≥15 pN. The rate for E537K, which is the same as that of WT at 5 pN, drops below zero at 50 pN, whereas the WT averages ~20 bp s −1 . Above 30 pN, the percent time packaging for all the mutants drops clearly below that of WT, and at 60 pN it drops to 0% for all the mutants versus ~12% for WT. At 50 pN the mutants displayed only brief episodes of highly slowed packaging, and at 60 pN no packaging was detected, whereas the WT motor was still able to package with an average motor velocity of ~100 bp s −1 . 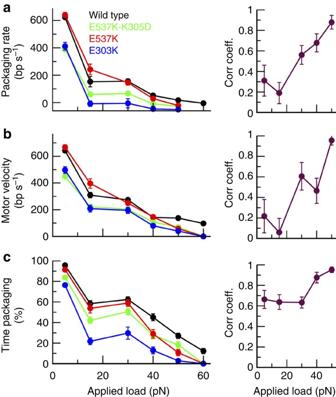Figure 3: Experimental metrics of motor activity and correlation with computed free-energy changes in gp17. (a–c, left panel) Average measured packaging rate (a), motor velocity (b) and % time spent packaging (c) detected in 1-s time intervals for WT gp17 (black), E537K (red), E537K-K305D (green), E303K (blue). The number of independent packaging events measured for each complex is given inSupplementary Table 1, and the error bars indicate s.e.m. (a–c, right panel) Corresponding Pearson correlation coefficients (min=0, max=1) between experimental metrics of motor function (adjacent plots) and calculated free-energy changes between the extended and compact forms of gp17. The error bars indicate s.e.m. Figure 3: Experimental metrics of motor activity and correlation with computed free-energy changes in gp17. ( a – c , left panel) Average measured packaging rate ( a ), motor velocity ( b ) and % time spent packaging ( c ) detected in 1-s time intervals for WT gp17 (black), E537K (red), E537K-K305D (green), E303K (blue). The number of independent packaging events measured for each complex is given in Supplementary Table 1 , and the error bars indicate s.e.m. ( a – c , right panel) Corresponding Pearson correlation coefficients (min=0, max=1) between experimental metrics of motor function (adjacent plots) and calculated free-energy changes between the extended and compact forms of gp17. The error bars indicate s.e.m. Full size image Thus, the mutant motors exhibit a reduced force-generation capacity, with F max between 50 and 60 pN. Overall, these results showed that all of the charged residues altered by mutagenesis play an important role in motor function. These results are consistent with the electrostatic force model because residue changes expected to weaken the electrostatic interactions proposed to drive the extended-to-compact transition indeed cause impairments in the packaging rate and force-generating capacity of the motor. MD-based free-energy calculations We next sought to investigate more quantitatively how different residue changes would be expected to affect the conformational change of gp17 from the extended-to-compact states. In particular, we investigated whether the predicted degree of impairment would follow a similar trend as observed in our experimental measurements of impaired function, which increased in the following order: WT, E537K-K305D, E537K and E303K. To this end, we carried out MD simulations of gp17 to predict the free-energy difference Δ G EC between the extended ( E ) and compact ( C ) states observed in the structural studies. Because of the limited structural information for this system, we do not attempt to model the motor–DNA interaction or the full ATP hydrolysis cycle. Thus, our modelling is necessarily more limited compared with the more intricate models that have been developed to understand detailed structure–function relationships for other biomotors such as the large tumour antigen helicase and F1-ATPase, where structures are available in different nucleotide states and for the helicase with DNA bound [25] , [26] . We determined Δ G EC = G C − G E by computing the free energies of the compact ( G C ) and extended states ( G E ) relative to a common reference state. The relative free energies for each state were calculated as ‘binding free energies’ between the N- and C-terminal domains using the Molecular Mechanics Generalized Born Surface Area (MM-GBSA) approach [39] . In these calculations, the compact state was modelled as the available crystal structure of gp17 in the compact state, while the extended state observed in cryo-EM studies was modelled from the crystal structure by imposing a 7 Å separation between the N- and C-terminal domains. Our calculations yielded Δ G EC =−38.21±4.42 kcal mol −1 for WT gp17, −19.95±9.99 kcal mol −1 for E537K-K305D, −6.14±3.44 kcal mol −1 for E537K, and −2.79±5.55 kcal mol −1 for E303K. These values do not include contributions from changes in the configurational (mostly vibrational) entropy of the gp17, as we found that estimates of vibrational entropy from normal mode calculations yielded large uncertainties. We do not, however, expect vibrational entropy to vary significantly across different mutants. Notably the determined free-energy values are all negative, consistent with the transition from the extended-to-compact state being most favourable for the WT gp17 and favourable to a lesser degree for the mutants. We also carried out calculations for the mutant E309K, which exhibited no packaging activity in both bulk packaging assays and optical tweezers assays. Notably for this mutant we calculated a positive or near zero (unfavourable) Δ G EC =1.83±10.3 kcal mol −1 . For WT gp17, the calculated absolute value |Δ G EC | ≅ 38 kcal mol −1 is equivalent to ~260 pN·nm of energy, which would imply that the maximum force that can be exerted during the Δ x =0.7 nm separation change between the N- and C-terminal subdomains is F max =|Δ G EC |/Δ x ≅ 370 pN. Thus, our calculations show that the extended-to-collapsed state transition can indeed produce more than enough force to explain the very high measured forces (>60 pN) generated during packaging. The energy released by hydrolysis of one ATP under the experimental conditions is also sufficient to generate 60 pN of force, as discussed previously [14] . However, the predicted |Δ G EC | is about twice the ~130 pN·nm free energy released by hydrolysis of a single ATP molecule, suggesting hydrolysis would not provide enough energy to return from the compact state to the extended state. However, several caveats regarding the calculations could potentially be responsible for this discrepancy. Owing to lack of detailed structural information, we approximate the extended state structure by simply displacing the centre-of-mass of the C-terminal domain away from that of the N-terminal domain by 7 Å. In reality, changes in orientations of the domains may affect Δ G EC values [40] . Also, our calculations ignore the other components of the motor complex—neighbouring gp17 subunits along with the threaded DNA molecule—whose configuration remains undetermined. These components likely occlude portions of the N- and C-terminal domain interface from getting solvated, causing our calculations to either over- or under-predict the solvation free energy. Our calculations neglect potential contributions from the configurational entropy of gp17 within the full pentameric active complex, as discussed above. Finally, the MM-GBSA approach itself contains several approximations that may introduce inaccuracies in the absolute free energies values [41] and, like all other biomolecular simulations, our calculations are also subject to the inherent inaccuracies in the force field representation of protein, solvent and ions. For these reasons, we expect the relative trend of changes in Δ G EC with residue changes to be more meaningful than absolute Δ G EC values. Correlation of measured and computed impairments To compare the measured and calculated metrics of motor function we calculated the Pearson correlation coefficients (0=‘no correlation’, 1=‘perfect correlation’) between each of the three measured quantities ( Fig. 3 , right panel), at each of the five increasing values of applied force, and the calculated Δ G EC values for the WT gp17 and three mutants. We observe significant correlations in all cases and the degree of correlation increases with increasing applied force. At 5 pN, the packaging rate and motor velocity correlate only weakly with Δ G EC , but the correlation coefficients increase to 0.88 and 0.96, respectively, at 50 pN. The correlation coefficient for time spent packaging also rises from 0.65 to 0.95 as the force is increased from 5 to 50 pN. Thus, we have shown that the measured degree of motor impairment due to the residue changes correlates well with the calculated degree of impairment in terms of change in free-energy difference between the extended and compact states of gp17. The strength of correlation increases at high force, where the motor is subject to higher load, consistent with the proposal that the E-C transition is responsible for force generation. Several features, such as the double mutant E537K-K305D exhibiting less impairment than single mutant E303K, are reconciled by these calculations. The measured % times spent packaging and motor velocities also asymptote towards zero with increasing force in the order E303K, E537K, E537K-K305D and WT, consistent with the order of increasing magnitudes of the calculated favourable free-energy changes. Mechanochemical energy landscape model Based on our findings above, we propose a minimal free-energy landscape model of gp17 mechanochemistry ( Fig. 4 ) that provides additional insights into the dynamics of the phage T4 DNA packaging motor. As discussed before, we do not attempt to model the motor–DNA interactions because of the lack of structural information. In this model, the free-energy landscape ( G tot ) governing gp17 motor function under applied loads is made up of contributions from the intrinsic conformational free-energy landscape of gp17 ( G gp17 ), the chemical free energy of ATP during the hydrolysis cycle ( G ATP ), and the mechanical work performed by gp17 against the applied load during DNA translocation ( W ), that is, G tot = G gp17 + G ATP + W . 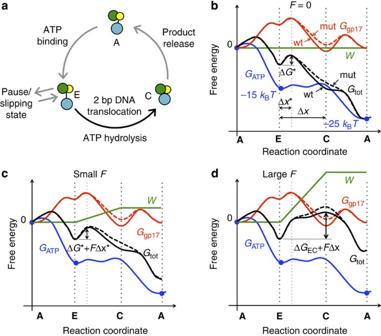Figure 4: Mechanochemical energy landscape model inferred from experimental and computational findings. (a) Proposed coupling between conformational transitions in gp17 and chemical transitions in ATP during a 2-bp DNA translocation cycle driven by the hydrolysis of one ATP molecule. The pausing and slippage of DNA is represented as an alternative state branching off from and rejoining at the extended state of gp17. (b–d) The conformational energy landscape of gp17 (red line), the ATP hydrolysis free-energy profile (blue line) and mechanical work (green line) add up to yield the overall mechanochemical energy landscapes (black line). The shapes of the different energy landscapes are schematically drawn for three cases: zero load (b), small load (c) and large applied loads (d). Figure 4: Mechanochemical energy landscape model inferred from experimental and computational findings. ( a ) Proposed coupling between conformational transitions in gp17 and chemical transitions in ATP during a 2-bp DNA translocation cycle driven by the hydrolysis of one ATP molecule. The pausing and slippage of DNA is represented as an alternative state branching off from and rejoining at the extended state of gp17. ( b – d ) The conformational energy landscape of gp17 (red line), the ATP hydrolysis free-energy profile (blue line) and mechanical work (green line) add up to yield the overall mechanochemical energy landscapes (black line). The shapes of the different energy landscapes are schematically drawn for three cases: zero load ( b ), small load ( c ) and large applied loads ( d ). Full size image We consider the simplest ‘tight coupling’ model in which ATP hydrolysis is assumed to result in one DNA translocation step. The energetics of ATP hydrolysis by motors with structurally homologous ATPase domains has been well characterized and has been shown to consist of two main steps that release energy: the ATP binding and product release steps [24] . The approximate G ATP profile based on ref. 24 is sketched as the blue line in Fig. 4b–d ; in these conditions, the ATP binding and product release steps yield ~15 k B T and ~10 k B T energies, respectively. We propose a minimal model consisting of three conformational states of gp17 ( Fig. 4a ). Before ATP binding, gp17 is in an Apo state ( A ) whose structure is not known. In the first step, ATP binds and provides the energy to drive the transition from the Apo state to the extended state ( E ), whereupon it engages the DNA. In the second step, ATP is hydrolyzed to ADP and P i and gp17 transitions from the extended state to the compact state ( C ), and translocates the DNA by 2 bp. In the third step, ADP and P i are released and the DNA is passed onto the next gp17 subunit in the motor ring (alternatively, P i could be released earlier during the second step, as suggested by studies of the phage φ 29 motor [17] ). The original gp17 subunit goes back to the A state. This order of conformational–chemical transitions allows for the E → C transition—that goes ‘downhill’ in free energy, as observed from our free-energy calculations, and requires no external energy—to occur during the ATP hydrolysis step that itself releases little or no energy [24] . This then allows for the ATP binding and product release steps, the two energy-producing chemical transitions, to be utilized for pushing gp17 towards the energetically unfavourable extended state ( A → E ) and releasing gp17 from its energetically favourable compact state ( C → A ), respectively. This proposed G gp17 profile is shown in Fig. 4b–d as the red line. Note that based on our simulations we only know that G gp17 decreases during the E → C transition, with free-energy difference Δ G EC ≡ G gp17 ( C )— G gp17 ( E )<0, and increases during the A → E and C → A transitions, possibly involving energy barriers, but the magnitudes of the free-energy differences and the heights and locations of the energy barriers are not known. The mechanical work W is given by the applied force F multiplied by the distance the DNA is translocated against the force. During the A → E transition, W =0, as there is no DNA packaging during this transition. During the E → C transition, W = F · x , where x is the distance the DNA moves during this transition. At the end of this transition, the net amount of work performed is W = F ·Δ x , where Δ x =2 bp. No additional work is performed during the C → A transition, and the work remains at W = F ·Δ x . The resulting W profile is shown as the green line in Fig. 4b–d . In the absence of a load force ( Fig. 4b ), the overall free-energy profile G tot (shown as the black line) exhibits a largely downhill path, potentially with energy barriers between each of the three conformational transitions, which facilitates efficient packaging of DNA. As described earlier, this is made possible by the constructive coupling between conformational and chemical transitions, which allows for efficient utilization of the energy released from ATP hydrolysis. Overall, each DNA translocation step of 2 bp leads to a net reduction in the free energy of the system (gp17+solution) equal to the total free energy released by the hydrolysis of one ATP molecule, that is, Δ G ATP ≅ 25 k B T . The observed reduction in the motor velocity with increasing load force F ( Fig. 3b ) suggests the presence of an energy barrier between the E and C states. The applied force, due to the mechanical work W , increases this barrier height by an amount ~ F ·Δ x *, where Δ x * is the location of the barrier relative to the E state along the force direction. Assuming an Arrhenius-like dependence in transition rates across barriers [38] , the DNA translocation rate k t (and hence the motor velocity) should then approximately decrease with increasing F via k t ∝ ~exp[−(Δ G * + F ·Δ x *)/ k B T ], where Δ G * denotes height of this energy barrier ( Fig. 4c ). However, based on our findings with gp17 mutants we propose that at sufficiently large F , the work term tilts the energy landscape between E and C states to such a large extent that the free energy of state C now becomes higher than that at the original barrier, making the crossing of state C the rate-limiting step ( Fig. 4d ). The relevant barrier height then becomes equal to the free-energy difference between states E and C , as given by Δ G EC + F ·Δ x . The rate of DNA translocation should consequently reduce via k t ∝ ~exp[−(Δ G EC + F ·Δ x )/ k B T ]. Our measurements show that the mutant motors generate smaller packaging forces than WT motors. This effect can be understood based on our free-energy calculations, which predict the E → C transition as being less favourable for mutants, leading to larger state C free energies for the mutants as compared with the WT motor, as depicted in Fig. 4b–d . In addition to having lower stall forces (<60 pN), the mutants also exhibit slower rates of packaging as compared with WT motors, and this difference becomes more significant at high loads. This can be explained by our model, which predicts that the rate of DNA translocation varies as k t ∝ exp[−(Δ G *+ F ·Δ x *)/ k B T ] at low loads and as k t ∝ exp[−(Δ G EC + F ·Δ x )/ k B T ] at high loads. That the mutants and WT motors exhibit smaller differences at low forces implies that they both exhibit similar energy barriers Δ G * ( Fig. 4c ). In contrast, the stronger effect of mutations on the packaging rate at high loads is consistent with the mutations decreasing the magnitude of Δ G EC ( Fig. 4d ). The observed increase in pausing and slipping of DNA during translocation with high applied force and with mutations ( Fig. 2 ) can also be explained by the energy landscape model. A recent study of T4 packaging at low ATP concentration suggested the presence of a pause-‘unpackaging’ state in the mechanochemical kinetic cycle that branches off from the DNA translocation pathway [42] . Our present results further suggest that with saturating ATP the motor can switch to this alternate pathway while residing at the E state under a high load force, which represents the most stretched conformation of the motor ( Fig. 4a ). It then follows that conditions slowing down the E → C transition rate, such as the applied load and the residue changes studied here, would increase the time that the motor resides in the E state. This in turn increases the chances of the motor entering the proposed pause-unpackaging state, leading to increased rates of pausing and slipping, which is consistent with our observations. Using a combination of single-molecule measurements with applied forces, site-directed mutagenesis and MD simulations, we have quantitatively demonstrated the importance of electrostatic interactions between residues located at the interface of the N- and C-terminal subdomains of gp17 to mediate DNA translocation. These findings support the T4 motor force-generation mechanism proposed by Sun et al. [27] on the basis of structural data. We show that our results with both WT and mutant motors under a wide range of load forces can be rationalized, at least qualitatively, by an energy landscape model that couples the free-energy profile of motor conformational states with that of the ATP hydrolysis cycle. Many molecular motors rely on large-scale structural rearrangements to forcibly translocate cargo. These rearrangements are often coupled to structural changes in the vicinity of the ATP-binding pocket during the ATP hydrolysis cycle, which cause allosteric effects that may be leveraged to produce large-scale motions. Although coordination of multiple parallel electrostatic interactions across an interface between two subdomains has not been previously demonstrated as a mechanism to directly produce motor force, evidence suggests that both myosin [43] and FoF1-ATP synthase [44] rely on electrostatic interactions between single pairs of charged residues to initiate structural transitions largely mediated by polar and hydrophobic interactions. As the T4 motor shares some features with many other ring-shaped nucleoside triphosphatases, including enzyme complexes involved in DNA replication and transcription (helicases), protein degradation and chromosome segregation, the force-generation mechanism investigated here may well have broader implications [45] . Materials A 25,339-bp dsDNA construct used as a substrate for packaging was prepared by PCR from lambda phage DNA (NEB, Inc.) using primers biotin-5′-CTGATGAGTTCGTGTCCGTACAACTGGCGTAATC-3′ and 5′-ATCCGATCTGCGTTACCGAATGGATGGATG-3′ (Operon, Inc.) and the PCR Extender System (5 Prime, Inc.) [37] . T4 phage heads were purified from the 10am.13am.hoc-del.soc-del phage mutant [46] , [47] . E. coli P301 (sup−) cells infected with this mutant were lysed in Pi-Mg buffer (26 mM Na 2 HPO 4 , 68 mM NaCl, 22 mM KH 2 PO 4 , 1 mM MgSO 4 , pH 7.5) containing 10 μg ml −1 DNase I and chloroform and incubated at 37 °C for 30 min. The lysate was subjected to two low- (6,000 g for 10 min) and high-speed centrifugations (35,000 g for 45 min) and the final heads pellet was resuspended in Tris–Mg buffer (10 mM Tris–HCl, pH 7.5, 50 mM NaCl and 5 mM Mg Cl 2 ) and purified by CsCl density gradient centrifugation. The major head band sedimented at about one-third from the bottom of a 5 ml gradient was extracted and dialyzed overnight against Tris–Mg buffer. The heads were further purified by DEAE-Sepharose ion-exchange chromatography. The peak heads fractions were concentrated and stored at −80 °C. WT and mutant gp17 motor proteins were purified from E. coli BL21 (DE3) RIPL cells harbouring the recombinant clones [46] , [47] . The recombinant proteins were over-expressed with 1 mM IPTG for 2 h at 30 °C. The cells were harvested by centrifugation (4,000 g for 15 min at 4 °C) and resuspended in HisTrap-binding buffer (50 mM Tris–HCl, pH 8.0, 20 mM imidazole and 100 mM NaCl). The cells were lysed using French-press (Aminco, USA) and the soluble fraction containing the His-tagged fusion protein was isolated by centrifugation at 34,000 g for 20 min. The supernatant was loaded onto a HisTrap column (GE Healthcare), washed with 50 mM imidazole containing buffer and the protein was eluted with 20–500 mM linear imidazole gradient. The peak fractions were concentrated and purified by size exclusion chromatography using Hi-Load 16/60 Superdex-200 (prep-grade) gel filtration column (GE Healthcare) in a buffer containing 20 mM Tris–HCl, (pH 8.0) and 100 mM NaCl. The peak fractions were concentrated and stored at −80 °C. Bulk DNA packaging assays DNase protection assays shown in Supplementary Fig. 2 were performed as follows [48] . The purified WT or mutant gp17 proteins were incubated with phage heads in the presence of 30 mM Tris–HCl (pH 7.5), 100 mM NaCl, 3 mM MgCl 2 , 1 mM ATP and phage λ DNA (48.5 kb) for 30 min at 37 °C. DNase I (Sigma) was added to terminate DNA packaging and digest the unprotected DNA. Proteinase K (0.5 μg μl −1 ), 50 mM EDTA and 0.2% SDS were added and incubated for 30 min at 65 °C to digest DNase I and capsid and release the packaged DNA. The samples were electrophoresed on 0.8% (w/v) agarose gel for 2–3 h at 100 V and DNA was stained with ethidium bromide. Single-molecule packaging measurements T4 head–motor complexes were prepared by mixing 1.7 × 10 10 heads with 70 pmol of gp17 in a solution containing 50 mM Tris–HCl (pH 7.5), 5 mM MgCl 2 , 80 mM NaCl, 1 mM gamma-S-ATP (non-hydrolyzable ATP analogue) and 450 ng of 120 bp ‘initiating’ DNA (which we found stabilizes the competent head–motor complex) [14] . This solution was incubated at room temperature for 45 min. Two microlitres of T4 antibody-coated 2.2-μm-diameter protein-G microspheres (Spherotech) were mixed with 10 μl of these stalled T4 complexes and incubated at room temperature for 45 min. The biotinylated dsDNA was attached to 2.2-μm-diameter streptavidin-coated microspheres (Spherotech). Measurements were carried out in solution containing 50 mM Tris–HCl (pH 7.5), 5 mM MgCl 2 , 80 mM NaCl, 1 mM ATP and 0.05 g l −1 BSA. High force measurements Packaging was first measured at low force (5 pN) for 5–10 s in force-clamp mode [14] to verify motor activity. The force was then quickly ramped (within 0.2 s) to a higher value by adjusting the set-point on the force-clamp control system. DNA translocation (packaging and/or slipping) was then tracked in force-clamp mode until the DNA tether was lost. The force was monitored at 2 kHz and was held constant by a feedback control system that adjusts the separation between the two traps in 0.5-nm increments. The optical tweezers system was calibrated as described previously [49] , [50] . Data analysis The motor velocity was calculated using methods similar as those described previously [14] by linear fitting of the DNA length versus time records in a 1-s sliding window. Slips larger than 100 bp and pauses in which the velocity dropped to <12 bp s −1 in the 1-s window were not included in determining ‘motor velocity’ (but were included in determining overall ‘packaging rate’). Free energy calculations Our aim is to compute the free-energy difference Δ G EC ≡ G C − G E between the extended and compact states of gp17 for the WT and mutant proteins. In principle, Δ G EC can be computed from all-atom MD simulations via approaches like umbrella sampling, though such approaches would entail prohibitive computational costs for systems as large as gp17. To this end, we use the MM-GBSA method [39] , which provides quick estimates of the binding free energy of molecular complexes by approximating the solvation free energy using implicit solvent mean field models. However, the application of MM-GBSA to computing intramolecular binding free energies, as opposed to intermolecular binding free energies, requires the N- and C-terminal domains to be treated as separate ‘molecules’, which assumes, consistent with structural features observed in ref. 27 , that the hinge joining the two domains is flexible and does not contribute much to the free-energy difference between the compact and extended states. One can then obtain Δ G EC using the free-energy cycle shown in Supplementary Fig. 3 , where the MM-GBSA method is used to compute the binding free energies Δ G bind,E and Δ G bind,C for assembling the N- and C-terminal domains into extended and compact states from a common isolated state in which the two domains do not interact with each other. The required free-energy difference can then be simply calculated as Δ G EC =Δ G bind,C −Δ G bind,E . Preparation of initial configurations The MM-GBSA method involves all-atom MD simulations of the extended and compact state complexes in explicit solvent and ions, starting from suitable initial configurations. These initial configurations were prepared based on the high-resolution crystal structure of gp17 in the compact state (PDB code: 3CPE) [27] . To generate the initial configuration of the compact state complex, we solvated the crystal structure in a TIP3P water box extending 10 Å from the surface of the protein in each direction by using the solvate function in VMD and then added 150 mM NaCl by using the autoionize function in VMD [51] . The solvated structure was energy minimized using 100 steps of steepest gradient, and then equilibrated using MD simulations for 0.5 ns to yield the initial configuration of the compact state complex. The atomic structure of the extended state is not known from X-ray studies but the cryo-electron microscopy studies show that the C- and N-terminal domains are spaced a further ~7 Å apart as compared with the compact state [27] . To generate an atomic model of this state we generated a vector between the centre of mass of the N- and C-terminal domains and used steered MD simulations to pull the C-terminal domain along this vector at a slow rate of 0.0002 Å fs −1 until a separation of 7 Å between the two centre of masses was achieved. The resulting structure was equilibrated using MD simulations for 0.5 ns. To generate the extended and compact state complexes for the three studied mutants, we used the mutator function in VMD to replace the chosen residue with the desired residue in the final equilibrated complexes. We then carried out 100 steps of energy minimization via steepest descent to allow the mutated residue as well as the nearby residues and water molecules to relax to their low-energy conformations. Energy minimization and MD simulations used for preparing the initial configurations were performed in NAMD [52] using the CHARMM 27 force field [53] . The simulations were carried out at constant temperature and pressure consistent with physiological conditions. The temperature was maintained at 310 K using a Langevin thermostat with a damping constant 1 ps −1 and the pressure was maintained at 1 atm using a Langevin piston with a period of 100 fs and damping time constant of 50 fs. We used a time step of 2 fs for integrating the equations of motion and employed the SHAKE algorithm to constrain all bond lengths involving hydrogen atoms. For computing short-range non-bonded interactions, a cutoff distance of 12 Å was employed. The simulations were carried out with periodic boundary conditions with all electrostatic interactions computed using the particle mesh Ewald method with grid spacing of 1 Å. We generated three additional initial configurations of the complexes by performing MD simulations of the original initial configurations described above. These additional simulations were carried out at three different temperatures (300, 320 and 330 K) for 50 ps while imposing a weak restraint on all heavy atoms of the protein via a harmonic potential with a spring constant of 2.0 kcal mol −1 Å −2 . This procedure forced the configurations to depart significantly from the starting configuration while remaining stable at these non-physiological temperatures. We carried out a further 600 ps of MD simulations during which the restraints were removed and the temperatures were brought back to 310 K. Thus, a total of four different initial configurations for each complex were obtained, allowing us to carry out four independent MM-GBSA calculations for improving the accuracy of our free-energy estimates. MM-GBSA calculations We next performed exhaustive MD simulations of extended state and compact state complexes for WT and mutant gp17. The binding free energies Δ G bind,E and Δ G bind,C were computed according to MM-GBSA via the following relation: Δ G bind =Δ E MM +Δ G solv − T Δ S conf , where Δ E MM , Δ G solv and T Δ S conf represent respective changes in molecular mechanics energy, solvation free energy and configurational entropy of the C- and N-terminal domains as they associate into a complex (extended or compact). The three free-energy contributions were computed from 500 snapshots of each complex recorded during 4 ns MD simulations, carried out using the mm_pbsa.pl script in AMBER 10 (ref. 54 ). In these calculations, we defined the N- and C-terminal domains as separate molecules, namely, the ‘receptor’ and ‘ligand’, respectively, and the full-length gp17 molecule as the ‘complex’, as explained earlier. Since the flexible hinge region contains residues 358–362, we define the N- and C-terminal domains by residues 1–359 and 360–560, respectively. The Δ E MM contributions were directly computed as the change in the sum of the bonded, electrostatic and vdW interaction energies. The Δ G solv contributions were further divided into polar and nonpolar contributions. The polar contributions were calculated using the Generalized Born approach [55] , [56] , while the nonpolar contributions were calculated from changes in solvent accessible surface area upon binding multiplied by the surface tension [34] . We used a water probe of radius 1.4 Å and a surface tension of 0.0072, kcal mol −1 Å −2 for the latter calculation. The T Δ S conf contributions are typically computed using normal mode analysis [35] , but these calculations were found to converge extremely slowly. Hence, we neglected its contributions to the free-energy difference. However, we believe that these entropic contributions will mostly cancel out when comparing Δ G EC values across WT and mutant gp17. The algorithms and associated parameters, force field and external conditions used for these MD simulations were kept identical to those used for generating the initial conditions. To obtain reliable values of Δ G EC as well as statistical uncertainties, we carried out four sets of MM-GBSA calculations for each WT and mutant complex, each starting from the four different initial configurations of the extended and compact state complex prepared using the procedures described in the previous section. How to cite this article: Migliori, A. D. et al. Evidence for an electrostatic mechanism of force generation by the bacteriophage T4 DNA packaging motor. Nat. Commun. 5:4173 doi: 10.1038/ncomms5173 (2014).